De novolipogenesis in human fat and liver is linked to ChREBP-β and metabolic health Clinical interest in de novo lipogenesis has been sparked by recent studies in rodents demonstrating that de novo lipogenesis specifically in white adipose tissue produces the insulin-sensitizing fatty acid palmitoleate. By contrast, hepatic lipogenesis is thought to contribute to metabolic disease. How de novo lipogenesis in white adipose tissue versus liver is altered in human obesity and insulin resistance is poorly understood. Here we show that lipogenic enzymes and the glucose transporter-4 are markedly decreased in white adipose tissue of insulin-resistant obese individuals compared with non-obese controls. By contrast, lipogenic enzymes are substantially upregulated in the liver of obese subjects. Bariatric weight loss restored de novo lipogenesis and glucose transporter-4 gene expression in white adipose tissue. Notably, lipogenic gene expression in both white adipose tissue and liver was strongly linked to the expression of carbohydrate-responsive element-binding protein-β and to metabolic risk markers. Thus, de novo lipogenesis predicts metabolic health in humans in a tissue-specific manner and is likely regulated by glucose-dependent carbohydrate-responsive element-binding protein activation. Lipid metabolism in white adipose tissue (WAT) and the liver contribute to whole-body metabolic homoeostasis [1] , [2] , [3] . Recent rodent studies demonstrated that de novo lipogenesis (DNL), the synthesis of fatty acids from non-lipid precursors, in WAT is downregulated in obesity and that restoring DNL selectively in WAT reverts obesity-dependent insulin resistance [4] , [5] , suggesting that reduction in DNL or alterations in the relevant products such as monounsaturated fatty acids is an important contributor to systemic insulin resistance and metabolic disease. Palmitoleate (C16:1n7), a DNL-derived fatty acid, appears to mediate the insulin-sensitizing effects of DNL in murine WAT [4] , [6] , [7] . In contrast to WAT, DNL in the liver has been found to be upregulated in rodent and human obesity, where it is believed to promote lipotoxicity, insulin resistance, non-alcoholic fatty liver disease (NAFLD) and atherogenic dyslipidemia [8] . Proposed molecular mechanisms of DNL-induced lipotoxicity are, for example, exaggerated synthesis of insulin resistance-inducing ceramides from palmitate (C16:0) (ref. 9 ) and activation of the innate immune system by saturated fatty acids [10] . Based on this association between hepatic DNL and the metabolic syndrome, it is believed that inhibition of DNL may be a viable approach to treating obesity-related disorders such as type 2 diabetes (T2D) (ref. 11 ). However, assuming that DNL in human WAT is associated with metabolic health, this may not be a promising approach when used systemically. Bariatric surgery has become an important therapeutic option for the treatment of severe obesity-associated insulin resistance and T2D. Weight loss after bariatric surgery increases insulin sensitivity in liver, muscle and fat [12] . Furthermore, it improves metabolic inflammation [13] , atherogenic dyslipidemia [14] as well as NAFLD (ref. 15 ). With regard to WAT function, bariatric surgery was reported to normalize lipolysis [12] and plasma levels of adipokines [16] . Thus, it is well recognized that bariatric surgery can improve overall metabolic health, but it remains unclear how it improves insulin sensitivity [17] , and whether DNL in WAT changes after bariatric surgery-induced weight loss. To explore the effect of obesity on WAT and liver DNL and the potential reversibility of obesity-induced DNL changes after bariatric weight loss, we analysed the expression of key DNL enzymes and regulators in visceral and subcutaneous WAT (SAT) as well as liver samples collected in two cohorts of metabolically well-characterized human subjects. Furthermore, we determined the fatty acid composition of WAT to study the potential impact of DNL-derived fatty acids on metabolic health. Finally, the relation of altered DNL in WAT and liver, respectively, to metabolic risk was investigated by determining the correlations of DNL proteins and fatty acids with measures of insulin resistance and NAFLD. Obesity is associated with reduced DNL in visceral WAT We assessed the effects of obesity on WAT DNL by mRNA expression analyses in visceral WAT (VAT) specimens of all 165 study subjects, focusing on four key enzymes: acetyl-CoA carboxylase (ACC) and fatty acid synthase (FASN), the enzymes converting acetyl-CoA to palmitate (C16:0) (ref. 18 ), stearoyl-CoA desaturase (SCD) that carries out Δ9-desaturation of saturated fatty acids such as the C16:0 conversion to C16:1n7 (ref. 19 ) and fatty acid elongase 6 (ELOVL6), which elongates C16 to C18 fatty acids [20] . FASN and ELOVL6 mRNA were downregulated in VAT of obese subjects, whereas SCD was increased, as demonstrated by a statistical model (analysis of covariance, ANCOVA) addressing the association of body mass index (BMI) with DNL gene expression and its relationship with age and gender ( Fig. 1a–c ). Within the model, the expression of FASN and SCD was independent of gender, whereas ELOVL6 expression was somewhat lower, and less dependent on BMI, in females ( Supplementary Table S1 ). Furthermore, the negative associations of BMI with FASN and ELOVL6 mRNA were exaggerated with higher age, as revealed by significant interaction terms: BMI × age in the ANCOVA model ( Supplementary Table S1 ). 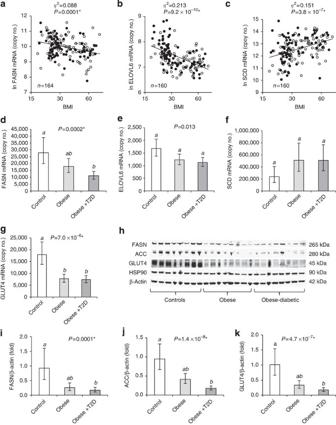Figure 1: Expression of metabolic and lipogenic genes in VAT of obese subjects. Log-transformed copy numbers of FASN (a), ELOVL6 (b) and SCD (c) mRNA in VAT plotted against BMI (logarithmic scale, non-logarithmic numbers), and group analysis comparing FASN (d), ELOVL6 (e), SCD (f) and GLUT4 (g) mRNA (n=19–21), as well as FASN (i), ACC (j) and GLUT4 (k) protein (n=14–17) in VAT of non-obese, obese and obese-diabetic (obese+T2D) subjects.a–c, open and closed circles are females and males, respectively. Trend lines as determined by ANCOVA including BMI as independent variable and gender as confounder are depicted as broken and solid lines for females and males, respectively. Effect size for BMI is described by partial eta-squared values (η2), describing the proportion of total variation attributable to BMI60. ANCOVA including age and interaction terms, seeSupplementary Table S1. (h) Representative VAT western blot.d–gandi–k, estimated marginal means with 95% confidence intervals as determined by ANCOVA. GLUT4 protein and mRNA levels were significantly higher in females compared with males (Supplementary Fig. S4). Groups identified by the same superscript letters (a,b) are not significantly different from each other (P≥0.0005). *Significant after adjustment for multiple testing. To account for the possibility that these apparent age effects were caused by an age bias inherent to the cohort, with obese subjects being on average much younger than non-obese, further detailed analyses were performed with three partially age-matched and fully gender-matched subgroups of the study population ( n =20; see Table 1 for anthropometric and clinical parameters). The control group consists of non-obese patients undergoing lower intestine surgery. The obese groups include obese bariatric surgery patients either without or with T2D, hereafter referred to as obese and obese-diabetic. Figure 1: Expression of metabolic and lipogenic genes in VAT of obese subjects. Log-transformed copy numbers of FASN ( a ), ELOVL6 ( b ) and SCD ( c ) mRNA in VAT plotted against BMI (logarithmic scale, non-logarithmic numbers), and group analysis comparing FASN ( d ), ELOVL6 ( e ), SCD ( f ) and GLUT4 ( g ) mRNA ( n =19–21), as well as FASN ( i ), ACC ( j ) and GLUT4 ( k ) protein ( n =14–17) in VAT of non-obese, obese and obese-diabetic (obese+T2D) subjects. a – c , open and closed circles are females and males, respectively. Trend lines as determined by ANCOVA including BMI as independent variable and gender as confounder are depicted as broken and solid lines for females and males, respectively. Effect size for BMI is described by partial eta-squared values (η2), describing the proportion of total variation attributable to BMI [60] . ANCOVA including age and interaction terms, see Supplementary Table S1 . ( h ) Representative VAT western blot. d – g and i – k , estimated marginal means with 95% confidence intervals as determined by ANCOVA. GLUT4 protein and mRNA levels were significantly higher in females compared with males ( Supplementary Fig. S4 ). Groups identified by the same superscript letters ( a , b ) are not significantly different from each other ( P ≥0.0005). *Significant after adjustment for multiple testing. Full size image Table 1 Anthropometric, demographic and clinical parameters of the experimental subgroups. Full size table In keeping with our findings in the total cohort, VAT mRNA expression levels of FASN and ELOVL6 ( Fig. 1d ) were lower in both obese and obese-diabetic individuals compared to non-obese controls, whereas SCD mRNA showed a trend for higher expression in obese subjects ( Fig. 1f ). No significant associations with gender or age were observed. The insulin-sensitive glucose transporter GLUT4 is a protein of particular interest for DNL, because it is rate-limiting for shuttling the DNL substrate glucose into adipocytes. Previously, GLUT4 was shown to be downregulated in SAT of obese or diabetic subjects [21] . Consistent with these results, we observed that VAT GLUT4 mRNA was markedly downregulated in both obese groups ( Fig. 1g ). Importantly, these findings were confirmed at the protein level. The expression of GLUT4, FASN and ACC was substantially decreased in obese and obese-diabetic individuals, as assessed by western blot analysis in the exact same cohort ( Fig. 1h–k ). VAT DNL is linked to ChREBP- β and metabolic risk factors The observed strong regulation of VAT DNL proteins prompted us to study known transcriptional regulators of DNL and to check whether they were downregulated themselves. Gene expression of the lipogenic transcription factor sterol response element-binding protein-1 (SREBP1) was unaltered in VAT of obese compared with non-obese subjects ( Fig. 2a ). Another important lipogenic transcription factor is carbohydrate-responsive element-binding protein (ChREBP), which is activated by increased glucose flux [22] and, therefore, is intimately linked to GLUT4 function in adipocytes. Interestingly, the expression of ChREBP-β, a recently discovered short isoform correlating strongly with ChREBP activity [23] , but not that of the conventional full length isoform, now termed ChREBP-α, was markedly reduced in obese and obese-diabetic compared to non-obese controls ( Fig. 2b ). Overall, ChREBP-β expression levels were, however, much lower than those of ChREBP-α. 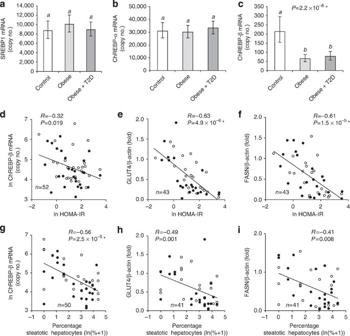Figure 2: VAT ChREBP-, FASN and GLUT4 are inversely linked to HOMA-IR and liver steatosis. Group analysis (n=17–21) comparing mRNA copy numbers of SREBP1 (a), ChREBP-α (b) and ChREBP-β (c) in VAT of non-obese, obese and obese-diabetic subjects. Pearson correlation analysis of VAT ChREBP-β mRNA (d,g), GLUT4 protein (e,h) and FASN protein (f,i) with HOMA-IR (d–f) and liver steatosis (g–i).a–c, estimated marginal means with 95% confidence intervals as determined by ANCOVA. Groups identified by the same letters (a,b) are not significantly different from each other (P≥0.0005). SREBP1 and ChREBP-β mRNA were significantly higher in females compared with males (Supplementary Fig. S4). *Significant after adjustment for multiple testing. Figure 2: VAT ChREBP-, FASN and GLUT4 are inversely linked to HOMA-IR and liver steatosis. Group analysis ( n =17–21) comparing mRNA copy numbers of SREBP1 ( a ), ChREBP-α ( b ) and ChREBP-β ( c ) in VAT of non-obese, obese and obese-diabetic subjects. Pearson correlation analysis of VAT ChREBP-β mRNA ( d , g ), GLUT4 protein ( e , h ) and FASN protein ( f , i ) with HOMA-IR ( d – f ) and liver steatosis ( g – i ). a – c , estimated marginal means with 95% confidence intervals as determined by ANCOVA. Groups identified by the same letters ( a , b ) are not significantly different from each other ( P ≥0.0005). SREBP1 and ChREBP-β mRNA were significantly higher in females compared with males ( Supplementary Fig. S4 ). *Significant after adjustment for multiple testing. Full size image It was previously demonstrated that a reduced capacity for DNL in WAT is linked to insulin resistance in mice [4] , [23] . Furthermore, there is evidence that WAT DNL suppresses liver DNL and, consequently, reduces liver steatosis [4] . Therefore, we next asked whether the DNL-related molecules showing the strongest obesity-dependent regulation in VAT, namely ChREBP-β, FASN and GLUT4, were associated with insulin resistance and liver steatosis. Indeed, VAT GLUT4 protein, FASN protein and ChREBP-β mRNA correlated inversely with homeostasis model assessment of insulin resistance (HOMA-IR) ( Fig. 2d–f ) and the degree of liver steatosis ( Fig. 2g–i ). HOMA-IR and liver steatosis were, however, not independently associated with the DNL parameters, probably because they strongly correlate with each other ( R =0.67, P =1.4 × 10 −7 , Pearson correlation, two-tailed t -test). When both parameters were combined in an ANCOVA, only one of them showed a significant association, respectively, namely VAT ChREBP-β mRNA with liver steatosis, and VAT FASN and GLUT4 protein expression with HOMA-IR ( Supplementary Table S2 ). Regulation of DNL may differ between WAT depots and, although excessive SAT is believed to be less harmful than excessive VAT [24] , it is more abundant and this may have physiological implications. Therefore, we determined SAT DNL gene expression in all three experimental groups. Similar to VAT, we found a profound downregulation of FASN and GLUT4, but no significant regulation of ELOVL6 or SCD mRNA in SAT samples of obese and obese-diabetic subjects, whereas TNFα mRNA was upregulated in obese-diabetic subjects ( Fig. 3a–e ). ChREBP-α expression was decreased in SAT of obese-diabetic individuals ( Fig. 3f ), whereas ChREBP-β mRNA was detectable by PCR but expression was too low for quantification by real-time PCR ( Supplementary Fig. S1 ). 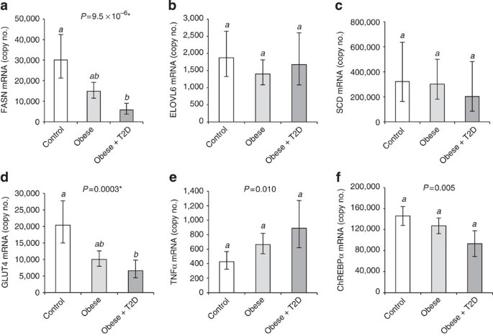Figure 3: SAT lipogenic gene expression in obese compared with non-obese subjects. Expression of FASN (a), ELOVL6 (b), SCD (c), GLUT4 (d), tumour necrosis factor-α (e) and ChREBP-α (f) mRNA in SAT. The subjects are a subset of the experimental groups described inTable 1. Numbers (female/male): controls (6/6), obese (9/10), obese-diabetic (2/5). Estimated marginal means with 95% confidence intervals, as determined by ANCOVA. Groups identified by the same letters (a,b) are not significantly different from each other (P≥0.0005). FASN, SCD and GLUT4 expressions were higher in females compared with males (Supplementary Fig. S4). *Significant after adjustment for multiple testing. Figure 3: SAT lipogenic gene expression in obese compared with non-obese subjects. Expression of FASN ( a ), ELOVL6 ( b ), SCD ( c ), GLUT4 ( d ), tumour necrosis factor-α ( e ) and ChREBP-α ( f ) mRNA in SAT. The subjects are a subset of the experimental groups described in Table 1 . Numbers (female/male): controls (6/6), obese (9/10), obese-diabetic (2/5). Estimated marginal means with 95% confidence intervals, as determined by ANCOVA. Groups identified by the same letters ( a , b ) are not significantly different from each other ( P ≥0.0005). FASN, SCD and GLUT4 expressions were higher in females compared with males ( Supplementary Fig. S4 ). *Significant after adjustment for multiple testing. Full size image Obesity is associated with less C18:0 but not C16:1n7 in VAT DNL in mice is tightly linked to the synthesis and abundance of C16:1n7 (ref. 4 ). In humans, C16:1n7 is believed to reflect Δ9-desaturase activity, that is, endogenous metabolism rather than diet [25] . To investigate whether decreased C16:1n7 could account for the insulin resistance in human obesity as described for mice [4] , [6] , [7] , we compared C16:1n7 concentrations in VAT of non-obese with those in obese and obese-diabetic subjects. VAT content of C16:1n7 was not diminished in obese subjects and only a moderate trend for a decrease was observed in obese-diabetic compared with obese ( Fig. 4a–d ). C16:1n7 concentration correlated positively with expression of both FASN and SCD in VAT ( Fig. 4e ). The fact that FASN and SCD are inversely altered in the obese state ( Fig. 1a ) may explain why C16:1n7 is not lower in human obesity. 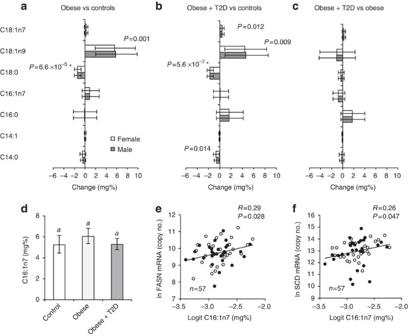Figure 4: VAT fatty acid concentrations are changed in obesity. Mean change (95% confidence interval) relative to total VAT fatty acids in obese versus controls (a), obese-diabetic versus controls (b), obese-diabetic versus obese (c). Estimated means and 95% confidence intervals of C16:1n7 (d) in controls, obese, obese-diabetic (n=15–21). Correlation of VAT C16:1n7 with mRNA expression of FASN (e) and SCD (f). Open bars and symbols are females;R, Pearson correlation coefficient. *Significant after adjustment for multiple testing. Figure 4: VAT fatty acid concentrations are changed in obesity. Mean change (95% confidence interval) relative to total VAT fatty acids in obese versus controls ( a ), obese-diabetic versus controls ( b ), obese-diabetic versus obese ( c ). Estimated means and 95% confidence intervals of C16:1n7 ( d ) in controls, obese, obese-diabetic ( n =15–21). Correlation of VAT C16:1n7 with mRNA expression of FASN ( e ) and SCD ( f ). Open bars and symbols are females; R , Pearson correlation coefficient. *Significant after adjustment for multiple testing. Full size image In contrast to C16:1n7, we detected a strong decrease in obese and obese-diabetic subjects for stearate (C18:0) ( Fig. 4a–c ) and very long chain-fatty acids derived from C18:0 (C20:0, C22:0, C24:0, C24:1, Supplementary Fig. S2 ). C16:0 was unchanged between groups ( Fig. 4a–c ). C18:0 trended to correlate positively with FASN ( R =0.21, P =0.13) and ELOVL6 expression ( R =0.27, P =0.04), but negatively with SCD ( R =−0.38, P =0.004) in VAT (Pearson correlations, two-tailed t -test). Thus, the decrease of FASN and ELOVL6 combined with the increase of SCD in VAT of obese patients might explain the reduction of VAT C18:0 in obesity. Next, we asked whether DNL-derived fatty acid species in VAT are linked to insulin resistance. C16:1n7 did not significantly correlate with HOMA-IR ( R =−0.14, P =0.33). By contrast, C18:0 demonstrated a strong, negative correlation comparable to those of the DNL proteins with HOMA-IR ( R =−0.50, P =0.00016), while oleate (C18:1n9) exhibited a positive but weaker correlation ( R =0.28, P =0.046; Pearson correlations, two-tailed t -test). SAT DNL gene expression is restored after bariatric surgery Bariatric surgery is a clinical intervention that often leads to marked weight loss and an improvement of metabolic health with the potential to cure T2D. The mechanisms mediating the salutary effects of bariatric surgery are not fully understood. To address the question whether increased WAT DNL may be one of them, we determined the expression of DNL genes in SAT obtained from obese patients before and after bariatric weight loss. As expected, bariatric surgery resulted in significantly reduced body weight and overall improvement of their metabolic state ( Table 2 ). Expression of FASN, ELOVL6 and GLUT4, but not SCD, in SAT increased after weight loss ( Fig. 5a–d ). Expression of ChREBP-α was moderately increased after weight loss ( Fig. 5e ), whereas ChREBP-β expression was below the level of detection. In contrast to upregulation of DNL, expression of TNFα was reduced after weight loss ( Fig. 5f ), which is consistent with a recent report [26] . Table 2 Anthropometric and clinical data of patients ( n =20) before and after bariatric intervention. 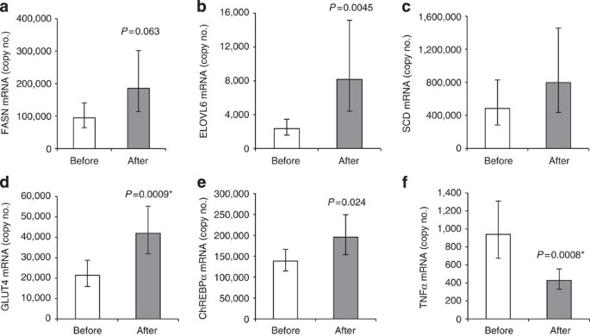Figure 5: Bariatric intervention increases expression of DNL-related genes and decreases tumour necrosis factor-α (TNF-α) expression in SAT. FASN (a), ELOVL6 (b), SCD (c), GLUT4 (d), ChREBP-α (e) and TNF-α (f) mRNA in SAT samples of bariatric surgery patients (n=16–20) before and after weight loss. Means and 95% confidence intervals, pairedt-test of log-transformed values. *Significant after adjustment for multiple testing. Full size table Figure 5: Bariatric intervention increases expression of DNL-related genes and decreases tumour necrosis factor-α (TNF-α) expression in SAT. FASN ( a ), ELOVL6 ( b ), SCD ( c ), GLUT4 ( d ), ChREBP-α ( e ) and TNF-α ( f ) mRNA in SAT samples of bariatric surgery patients ( n =16–20) before and after weight loss. Means and 95% confidence intervals, paired t -test of log-transformed values. *Significant after adjustment for multiple testing. Full size image Obesity is associated with increased liver ChREBP- and DNL Elevated liver DNL in obesity can contribute to the development of insulin resistance [8] . The role of liver DNL in metabolic disease in humans and especially its relationship to WAT DNL is, however, not well understood. Therefore we analysed DNL expression in liver biopsies of the exact same individuals having been used for analyses of VAT DNL. In contrast to VAT ( Fig. 1a–f ), we found that the mRNAs of FASN and ELOVL6 were significantly upregulated in livers of obese subjects ( Fig. 6a ; Supplementary Fig. S3a,b ). Liver SCD mRNA exhibited higher variability and a less pronounced increase in obese subjects ( Fig. 6c ; Supplementary Fig. S3c ). Liver FASN mRNA correlated inversely with VAT FASN protein ( Fig. 6g ), indicating a potential mechanistic link between VAT and liver FASN regulation in obesity. Regulation of DNL in liver was further studied by western blot analysis. Owing to sample limitations we were only able to analyse a small set of liver tissue specimens, different from the subgroups described in Table 1 (see Supplementary Table S3 ). FASN protein expression in obese subjects tended to be increased, although this analysis was underpowered, and we therefore failed to reach statistical significance in the ANCOVA ( Supplementary Fig. S3d ). FASN protein levels were, however, higher when both obese groups were combined and compared with the non-obese subjects ( Fig. 6h ) and they correlated with FASN mRNA quantified in the same liver specimens ( Supplementary Fig. S3f ), indicating that FASN mRNA levels reflect FASN protein levels in human livers. 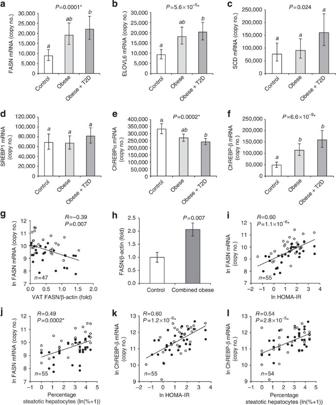Figure 6: Hepatic DNL is linked to higher BMI, HOMA-IR and liver steatosis. Group analysis (n=19–21) comparing liver mRNA expression of FASN (a), ELOVL6 (b), SCD (c), SREBP1 (d), ChREBP-α (e) and ChREBP-β (f) of non-obese, obese and obese-diabetic subjects. (a–f) Estimated marginal means with 95% confidence intervals as determined by ANCOVA. FASN mRNA is significantly higher in females compared with males (Supplementary Fig. S4). Groups identified by the same letters (a,b) are not significantly different from each other (P≥0.0005). Correlation of liver FASN mRNA with VAT FASN protein (g). FASN protein expression in non-obese subjects (n=13) compared with combined obese and obese-diabetic (n=15) (h), means±s.e.m., two-tailedt-test. Pearson correlation analysis of liver FASN mRNA (i,j) and liver ChREBP-β mRNA (k,l) with HOMA-IR (i,k) and liver steatosis (j,l). *Significant after adjustment for multiple testing. Figure 6: Hepatic DNL is linked to higher BMI, HOMA-IR and liver steatosis. Group analysis ( n =19–21) comparing liver mRNA expression of FASN ( a ), ELOVL6 ( b ), SCD ( c ), SREBP1 ( d ), ChREBP-α ( e ) and ChREBP-β ( f ) of non-obese, obese and obese-diabetic subjects. ( a – f ) Estimated marginal means with 95% confidence intervals as determined by ANCOVA. FASN mRNA is significantly higher in females compared with males ( Supplementary Fig. S4 ). Groups identified by the same letters ( a , b ) are not significantly different from each other ( P ≥0.0005). Correlation of liver FASN mRNA with VAT FASN protein ( g ). FASN protein expression in non-obese subjects ( n =13) compared with combined obese and obese-diabetic ( n =15) ( h ), means±s.e.m., two-tailed t -test. Pearson correlation analysis of liver FASN mRNA ( i , j ) and liver ChREBP-β mRNA ( k , l ) with HOMA-IR ( i , k ) and liver steatosis ( j , l ). *Significant after adjustment for multiple testing. Full size image Next, we asked whether the expression of lipogenic transcription factors was altered in livers of obese subjects in a fashion similar to their putative target genes. Liver mRNA levels of SREBP1 ( Fig. 6d ) were not increased in obesity. However, the expression of ChREBP-β was substantially elevated, whereas ChREBP-α was slightly decreased in livers of obese individuals ( Fig. 6e ), suggesting an important role for ChREBP-β in regulating liver DNL. In line with liver ChREBP-β and its target genes having a role in steatosis and potentially also with insulin resistance [8] , we observed a positive correlation of ChREBP-β and FASN mRNA with HOMA-IR and the degree of liver steatosis ( Fig. 6i–l ). The association with liver steatosis was, however, weaker and not independent of that with HOMA-IR ( Supplementary Table S2 ). In the present study we demonstrate that WAT DNL is suppressed in human obesity and T2D by showing that the expression of the key DNL enzymes ACC and FASN is markedly decreased in VAT of obese subjects. These findings are in line with previous publications reporting downregulation of lipogenic mRNAs in WAT of obese humans [27] , [28] , [29] and rodents [30] , [31] . In addition to the suppression of DNL enzymes, we observed a profound downregulation of GLUT4 in VAT of obese subjects ( Fig. 1 ), complementing previous studies that were limited to human SAT [21] , [32] . Moreover, we are the first to demonstrate a coordinated upregulation of WAT DNL genes and GLUT4 after bariatric weight loss ( Fig. 5 ). In light of transgenic mouse studies demonstrating that adipose tissue GLUT4 is an important regulator of whole-body insulin sensitivity [33] , the obesity-dependent GLUT4 decrease and the marked inverse correlation of GLUT4 protein with HOMA-IR observed in this study ( Fig. 2 ) strongly support the notion that GLUT4 promotes insulin sensitivity also in humans, possibly as a pacemaker of adipocyte DNL. GLUT4 does not only provide substrate for DNL, it is also critical for the lipogenic transcription factor ChREBP, which is activated on increased glucose flux [22] . Diminished ChREBP activation due to defective GLUT4 expression, and presumably GLUT4 translocation, may thus be responsible for the reduced DNL gene expression in obesity. While this manuscript was under preparation, a novel ChREBP isoform (ChREBP-β), derived from an alternative promoter, was described [23] . ChREBP-β is shorter than the conventional isoform (ChREBP-α) and has higher activity due to constitutive nuclear localization. We found a clear coregulation of ChREBP-β but not ChREBP-α with DNL genes in VAT ( Fig. 2 ). Our data, thus, complement the finding by Herman et al. [23] , which demonstrated a link of human SAT ChREBP-β to insulin sensitivity and GLUT4 expression. We did not observe a downregulation of the quantitatively dominant isoform ChREBP-α in VAT of obese subjects, as reported recently [34] , and only a moderate one in SAT ( Fig. 3 ). The discrepancy may be due to the younger age and the leaner phenotype of the non-obese controls in that study compared with ours. In addition to WAT, we show here for the first time that ChREBP-β is coregulated with DNL enzymes in liver ( Fig. 6 ). Given that the well-studied isoform ChREBP-α is regulated mostly at the posttranslational level, previous studies using gene expression readout could not reliably assess ChREBP activity. ChREBP-β mRNA levels better reflect activity because the ChREBP-β promoter is autoactivated by ChREBP [23] . Taken together, our data indicate that ChREBP regulates DNL in human liver, supporting the view that ChREBP, activated through elevated hepatic hexose flux, for example, by fructose-rich nutrition [35] or SREBP1-dependent induction of glucokinase [36] , is a major mechanism by which DNL is induced in livers of obese and insulin-resistant humans. Activity of DNL enzymes influences tissue fatty acid profiles [4] , [37] . We found that, in contrast to FASN, SCD was moderately upregulated in VAT of obese individuals ( Fig. 1 ). This suggests increased SCD activity in adipose tissue of obese individuals and can explain the most prominent fatty acid changes we observed in obese subjects, namely a decrease in C18:0 and an increase in C18:1n9 ( Fig. 4 ). Similarly, it may explain another important observation in our study, the lack of substantial obesity-dependent changes in VAT C16:1n7 concentration ( Fig. 4 ), which is consistent with a recent human study reporting a positive correlation of WAT C16:1n7 with BMI [38] . In obese mice, the murine SCD homologue SCD1 was found to be downregulated in WAT [4] , explaining the decrease of C16:1n7, but not C18:0 in all major lipid classes of WAT in these mice [4] . Thus, regulation of adipose tissue SCD seems to differ between humans and mice. Our data indicate a higher capacity of obese humans versus mice to adapt to an unhealthy excess of C18:0 and other saturated fatty acids through Δ9-desaturation. Although not studied in detail so far, there is some experimental evidence indicating that C18:0 in diet or as free fatty acid (FFA) induces insulin resistance [39] , [40] , [41] . Accordingly, the negative correlation of C18:0 with BMI and HOMA-IR that we and others [37] observed may rather reflect protective conversion of the unhealthy fatty acid C18:0 than a (hypothetical) insulin-sensitizing effect of C18:0. On the other hand, SCD1 and C18:1n9 were recently demonstrated to mediate obesity-induced inflammation and insulin resistance in WAT [42] . Thus, the observed induction of SCD in VAT of obese subjects can also be interpreted as a maladaptive state and it remains difficult to estimate the net effect on metabolic health. To what extent C16:1n7 is an insulin-sensitizing factor in humans, as it is in mice [4] , [6] , [7] , is a matter of ongoing debate [43] , [44] , [45] and cannot be directly inferred from our data. The current model assigns the insulin-sensitizing role to C16:1n7 within FFA, the major lipid class released from WAT [4] . For technical reasons, we did not measure fatty acids in the FFA fraction of VAT but determined total VAT fatty acid profiles. The latter closely correspond to serum FFA profiles in humans, at least with regard to C16:1n7 and other DNL-derived fatty acids [44] , [46] . In any event, the preserved concentration of C16:1n7 in VAT of obese subjects ( Fig. 4 ) may explain why C16:1n7 does not significantly correlate with HOMA-IR, in stark contrast to FASN and GLUT4 protein levels ( Fig. 2 ). It is conceivable that DNL-linked molecules other than FFA, which we may have missed in the total tissue fatty acid analysis, are released from adipose tissue and counteract insulin resistance. Clearly, more work is needed to unravel potential mechanisms connecting adipose DNL to systemic insulin sensitivity in humans, which may lead to the identification of alternative lipid species or non-lipid molecules with similar biological functions as C16:1n7 in rodents. In contrast to the downregulation of DNL in WAT we observed a profound induction of FASN, ELOVL6 and SCD in livers of obese subjects ( Fig. 6 ). This observation is very important as (i) it complements previous human studies that could assess hepatic DNL only indirectly through tracer incorporation into VLDL fatty acids [47] , [48] and (ii) it shows for the first time that there is an inverse correlation between liver and WAT FASN expression ( Fig. 6 ). The correlation of liver FASN expression with HOMA-IR and the degree of liver steatosis ( Fig. 6 ) supports the concept that hepatic lipogenic induction can promote the development of NAFLD and insulin resistance [8] . However, elevated liver DNL does not lead to insulin resistance in every case, as elegantly demonstrated in a recent study using adenoviral hepatic overexpression of ChREBP-α in mice. Despite massive liver triglyceride accumulation, these mice were not insulin resistant, and on high-fat diet even more insulin sensitive than controls [49] . Contrasting with these results, adenoviral ChREBP-α knockdown improved insulin resistance in leptin-deficient obese mice [50] . Furthermore, inducing DNL in liver through transgenic overexpression of SREBP1 induced insulin resistance in mice on normal diet [51] . Thus, excessive hepatic DNL does not invariably cause insulin resistance. Clearly, more research is needed to understand how disturbed liver lipid metabolism and patterns are linked to liver metabolic dysfunction [3] and whether DNL-linked steatosis in obese humans is cause or consequence of metabolic disease. At least, several rodent studies demonstrate that reducing the activity of DNL enzymes can be used to treat metabolic disorders. For example, it was reported that inhibiting liver FASN [11] or ELOVL6 (ref. 52 ) improved insulin resistance and atherosclerosis in mice. In light of these therapeutic proof-of-concept studies indicating beneficial effects on insulin resistance and atherosclerosis, our liver data provide important target validation for pharmacological DNL inhibitors. However, one needs to take into account that inhibition of these enzymes in WAT may promote systemic insulin resistance, as discussed above, and DNL inhibition with concomitantly reduced monounsaturated fatty acids may also have adverse effects in other cell types, especially in macrophages [53] and pancreatic β-cells [54] , [55] , [56] . Selective inhibition using molecules preferentially taken up by liver such as the FASN inhibitor platensimycin [11] could be a way to prevent unwanted consequences of DNL suppression in extra-hepatic tissues. As an additional measure, nutritional C16:1n7 supplementation could be used to mitigate negative effects of DNL inhibition. Given the strong effects of C16:1n7 on cultured macrophages and β-cells [53] , [54] , [55] , and positive results in mouse studies [6] , [7] , this is a promising approach that does, however, require in vivo validation studies in humans. In summary, our study demonstrates that DNL enzymes are markedly suppressed in WAT of obese subjects, as is GLUT4. This suppression is closely linked to impaired metabolic control and can be reversed by weight loss through bariatric intervention. Furthermore, we show that in obesity, liver DNL is profoundly upregulated, and is closely linked to insulin resistance as well as liver steatosis. Thus, DNL inversely correlates between WAT and liver and is closely linked with markers of metabolic health. The novel ChREBP isoform ChREBP-β is tightly associated with DNL gene expression in both VAT and liver, indicating a key role of glucose metabolism in the regulation of lipogenesis. Study subjects Patients undergoing bariatric surgery ( n =61), abdominal surgery for early colorectal cancer ( n =48), pancreatic cancer ( n =22), other cancers of the gastrointestinal tract or benign diseases such as sigma-diverticulosis at the Department of General and Visceral Surgery, University of Ulm, Germany, from 2002–2010 were included in the study. Exclusion criteria were type 1 diabetes and acute inflammatory disease. None of the cancer patients exhibited signs of metastases or reported excessive, unintended recent weight loss. Unlike in other bariatric centres, bariatric patients were not subjected to a weight loss regimen before surgery, but were commended to adhere to a regular meal pattern and take a multi-vitamin and mineral supplement 4 weeks before bariatric intervention, minimizing confounding effects of negative weight balance. Anthropometric and clinical data describing the study cohort are listed in Supplementary Table S4 . Surgical resection specimens, VAT, abdominal SAT, liver biopsies and blood were immediately placed on ice and subsequently snap-frozen in liquid nitrogen and stored in liquid nitrogen or at −80 °C. For detailed analyses, gender-matched subgroups including non-obese non-diabetic subjects (controls), obese non-diabetic subjects (obese) and obese subjects with T2D (obese-diabetic) were selected from the total cohort. To reduce the age gap between obese subjects (mostly morbidly obese, bariatric patients) and non-obese subjects (mostly cancer patients) the youngest obese patients (age <33 years) and the oldest non-obese patients (age >70 years) were excluded from the subgroups. Eventually, colorectal cancer ( n =15) and sigma-diverticulosis ( n =4) patients were selected as the control group. Most control subjects had no signs of overt inflammation, with only three individuals exhibiting elevated C-reactive protein (≥5 μg ml −1 , range 7.6–14.4 μg ml −1 ). See Table 1 for anthropometric and clinical data characterizing the subgroups. A separate population was used to investigate changes after bariatric surgery. Abdominal SAT resection specimens were obtained from 20 patients (15 females, 5 males) during bariatric surgery performed at Maastricht University Hospital, The Netherlands, from 2005–2010. Procedures were gastric bypass ( n =9), gastric banding ( n =4), gastric sleeve ( n =3), biliopancreatic diversion ( n =3) and Scopinaro ( n =1). Post-weight loss of abdominal SAT samples were taken from the same patients by excision 6 months ( n =7), 12 months ( n =10) or 24 months ( n =3) after bariatric surgery. All samples were taken in the fasted state and frozen immediately in liquid nitrogen before storage at −80 °C. Patients with type 1 diabetes, inflammatory diseases, and patients using anti-inflammatory drugs and/or reported alcohol consumption (more than 10 g per day) were excluded from the study. All blood samples were taken in fasted state before surgery and parameters were measured by routine methods in the clinical chemistry laboratories of Ulm and Maastricht University Hospitals. Liver steatosis (% of hepatocytes with visible lipid droplets) was estimated by the analysis of haematoxylin–eosin-stained liver specimens. In each case, permission was given from the local ethics committees in Maastricht, The Netherlands, and Ulm, Germany, and informed consent in writing was obtained from each subject. Gene expression analysis Total RNA was isolated and purified from tissue specimens using NucleoSpin RNA II kit (Macherey& Nagel). cDNA was synthesized using SuperScript III Reverse Transcriptase (Invitrogen). Quantitative real-time PCRs for indicated genes were performed on a 7900HT sequence detection system (Applied Biosystems) using TaqMan Assay-on-Demand primer-probe sets supplied by Applied Biosystems and selected to recognize all RefSeq sequences and a maximum of GenBank ESTs ( Supplementary Table S5 ). The ChREBP-α TaqMan assay (Hs00263027_m1) recognizes intron 1a. ChREBP-β expression was determined by SYBR green-based quantitative real-time PCR using an Mx3000P system (Stratagene) and primers as published [23] (forward: 5′-AGCGGATTCCAGGTGAGG-3′, reverse: 5′-TTGTTCAGGCGGATCTTGTC-3′). Gene expression was calculated as copy number per 10 4 copies of the housekeeper gene TATA binding protein-associated factor 1 (abbreviated as copy no.). Western blot analysis Protein extraction and western blot analysis were performed as described [57] . Briefly, frozen VAT (50–100 mg) or liver (30–50 mg) biopsies were homogenized in 20 mM MOPS, 2 mM EGTA, 5 mM EDTA, 30 mM sodium fluoride, 40 mM β-glycerophosphate, 10 mM sodium pyrophosphate, 2 mM sodium orthovanadate, 0.5% NP-40 and complete protease inhibitor cocktail (Roche) and centrifuged at 13,000 g for 20 min at either −3 °C (VAT) or +4 °C (liver). The supernatant was then collected while carefully avoiding the lipid layer on top and protein concentration was measured with a BCA protein quantification kit (Thermo Scientific). Protein extracts were separated on 4–12% NuPAGE gels (Invitrogen) and blotted onto Immobilon FL PVDF (Millipore) membranes. Membranes were blocked at room temperature for 1 h in Odyssey LI-COR Blocking Buffer (LI-COR) 1:2 diluted in TBS and incubated in primary antibodies in Blocking Buffer diluted 1:2 in TBS-T (0.1%) overnight at 4 °C. Primary antibodies against ACC (Cell Signaling Technology, dilution 1:1,000), FASN (BD Bioscience, 1:1,000), Hsp 90 (BD Bioscience, 1:1,000), β-actin (Abcam, 1:10,000), GLUT4 (Abcam, 1:2,000) and Hsc 70 (Santa Cruz Biotechnology, 1:10,000) were used. After three consecutive 5 min washes in TBS-T (0.1%), blots were incubated with Dylight 680-conjugated goat anti-rabbit IgG and Dylight 800-conjugated goat anti-mouse IgG (both Thermo Scientific) for 1 h at room temperature in blocking buffer containing 0.1% TBS-T and 0.1% SDS. After three washes in TBS-T and a final wash in TBS, the blots were scanned with the LI-COR Odyssey (LI-COR) and quantified with Odyssey 3.0 software based on direct fluorescence measurement. For quantification, proteins were normalized to β-actin. Fatty acid profiling Fatty acid composition in total lipid extracts of VAT was determined by gas chromatography, as described previously [58] . Briefly, 250 μl of butylhydroxytoluene (0.1 mol l −1 in methanol) and 6 ml of chloroform/methanol (2/1, v/v) were added to ~100 mg of tissue. After homogenization using an Ultraturrax homogenizer, the samples were heated to 50 °C for 30 min and centrifuged (1,800 g , 5 min). Fatty acid methyl esters were prepared by heating 100 μl of tissue extract, 2 ml methanol/toluene (4/1, v/v), 50 μl heptadecanoic acid (200 μg ml −1 in methanol/toluene, 4/1) and 200 μl acetylchloride in a capped tube for 1 h at 100 °C. After cooling to room temperature, 5 ml of 6% sodium carbonate and 1.6 ml of toluene were added. The mixture was centrifuged (1,800 g , 5 min) and 150–200 μl of the upper layer was transferred to auto sampler vials. Gas chromatography analyses were performed using an HP 5890 gas chromatograph (Hewlett Packard) equipped with flame ionization detectors (Stationary phase: DB-225 30 m × 0.25 mm i.d., film thickness 0.25 μm; Agilent). Peak identification and quantification was performed by comparing retention times and peak areas, respectively, to standard chromatograms. All calculations are based on fatty acid methyl ester values. Concentration of fatty acid species was calculated as mg% (mg fatty acid species/100 mg total fatty acids). Statistical methods Association of FASN gene expression with BMI in the whole cohort and apparent group effects were examined by ANCOVA, including gender and age as well as two-way interaction terms of independent variables in the initial models. Nonsignificant terms were hierarchically-backward eliminated as suggested by Kleinbaum and Klein [59] . Significant effects of age and gender are denoted in the results section when present. Bonferroni adjustment was applied in multiple group comparisons. To account for multiple testing, the threshold for statistical significance was set at P =0.05 divided by the number of statistical tests applied ( n =100, P <0.0005, main cohort; n =15, P <0.0033, bariatric intervention cohort). Paired t -tests were conducted to compare parameters before and after bariatric surgery. Data were transformed to natural logarithm when necessary to achieve normal distribution and/or homoscedasticity. Fatty acid concentrations were logit-transformed (ln[ x /(100– x )]). IBM SPSS Statistics version 19 was used for all statistical analyses. How to cite this article: Eissing, L. et al. De novo lipogenesis in human fat and liver is linked to ChREBP-β and metabolic health. Nat. Commun. 4:1528 doi: 10.1038/ncomms2537 (2013).